A thermoresponsive and chemically defined hydrogel for long-term culture of human embryonic stem cells Cultures of human embryonic stem cell typically rely on protein matrices or feeder cells to support attachment and growth, while mechanical, enzymatic or chemical cell dissociation methods are used for cellular passaging. However, these methods are ill defined, thus introducing variability into the system, and may damage cells. They also exert selective pressures favouring cell aneuploidy and loss of differentiation potential. Here we report the identification of a family of chemically defined thermoresponsive synthetic hydrogels based on 2-(diethylamino)ethyl acrylate, which support long-term human embryonic stem cell growth and pluripotency over a period of 2–6 months. The hydrogels permitted gentle, reagent-free cell passaging by virtue of transient modulation of the ambient temperature from 37 to 15 °C for 30 min. These chemically defined alternatives to currently used, undefined biological substrates represent a flexible and scalable approach for improving the definition, efficacy and safety of human embryonic stem cell culture systems for research, industrial and clinical applications. The use of pluripotent human embryonic stem cells (hESCs) in biomedical research and cellular therapies requires the development of efficacious and cost-effective defined culture systems for cell isolation, growth and differentiation. An important step to achieve these goals is the minimization or elimination of biological reagents which can be a source of pathogens and contribute to variable outcomes during cell processing. To date several feeder-independent and defined media formulations with the capacity to maintain both an undifferentiated hESC phenotype and cellular differentiation potential have been described [1] , [2] , [3] , [4] , [5] , [6] . These contain a broad range of proteins, lipids and small molecules that affect, amongst other things, intracellular signalling pathways controlling differentiation, and rely on extracellular matrix proteins such as laminin, fibronectin and vitronectin or protein-containing extracts [2] , [5] , [7] , [8] as substrates for cell attachment, with growth on such matrices typically being serum or albumin dependent [9] , [10] , [11] . Recently, polymer and peptide-polymer substrates have been reported with a capacity to sustain a hESC phenotype [12] , [13] , [14] , [15] , [16] . The limitations of these advances include variation in cell line responsiveness [15] and/or requirements for feeder cell conditioning of media or coating of surfaces with serum or serum proteins. Critically, for all substrates reported to date cell dissociation at passaging requires one or more treatments involving mechanical scraping or colony picking, proteolytic enzymatic digestion, or chemically mediated chelation of divalent cations (e.g., calcium and magnesium using EGTA or EDTA) [13] , [14] , [15] , [17] . Whereas mechanical dissociation is laborious and not readily scalable, enzymatic and chemical treatments can damage cells by removal of important surface proteins or ions (e.g., calcium) [18] , [19] . A promising alternative to reliance on mechanical, enzymatic or chemical release is binding and growth of cells on stimuli-responsive substrates which include polymers whose physical properties can be reversibly modulated by subtle changes in temperature or light. The utility of thermoresponsive polymers as substrates for cell binding and growth has already been established [20] , as has their use in contexts such as tissue engineering [21] , gene delivery [22] and reversible molecule absorption [23] , with cell dissociation from these substrates achieved by their swelling in response to the physical stimulus. Previously, we reported the fabrication of chemically defined polymers by inkjet printing [24] , [25] . In the current study, this method was used to identify combinations of acrylate and acrylamide monomers which generate chemically defined polymers that permit long-term maintenance of hESC and reagent-free dissociation in response to a reduction in ambient temperature. Polymer library screening Polymer arrays consisting of 609 different polymers spotted in quadruplicate [25] were synthesized in situ by inkjet printing mixtures of 18 monomers in seven different ratios in the presence of the crosslinker N , N ′-methylene bis acrylamide ( Supplementary Fig. S1 ). Monomers were chosen on the basis of their hydrophilicity, known tendency to permit modulation by temperature and pH, and their abilities to bind cells [25] , [26] . Array screening was performed in the biologically defined medium mTeSR1 ( [2] ). Our approach consisted of three phases of screening hESC for attachment to substrates before commitment to selected polymers for long-term culture ( Fig. 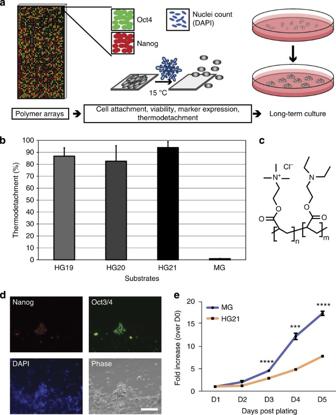Figure 1: Screening procedure for selection of polymers that support hESC culture. (a) Outline of the screening procedure used to select polymers that support hESC culture and passaging by thermodetachment. Cell attachment (nuclear count following DAPI stain), Oct3/4 and Nanog expression levels (immunocytochemistry) and thermodetachment ability (30 min at 15 °C) were assessed after culture of cells on polymer arrays. Successful polymers were selected for longer-term culture studies. (b) Cell detachment following lowering ambient temperature to 15 °C of hESC cultured on the top three polymers or Matrigel as control. Mean±s.d.,n=3. (c) Chemical structure of polymers HG19, 20 and 21 with 1:3, 1:1 and 3:1 ratios of AEtMA-Cl/DEAEA, respectively. (d) Following thermodetachment of RH1 hESC from HG21 the majority of the remaining cells, visualized by DAPI-stained nuclei (blue) and phase-contrast light microscopy, are negative for Oct3/4 (green) and Nanog (red) (immunocytochemistry). Scale bar, 100 μm. (e) Cell growth curves of RH1 hESC cultured on HG21 or MG, plotted as mean fold increase (±s.e.m.,n=3 biological replicates) relative to when cells were plated (day 0). ***P<0.001, ****P<0.0001 compared to D1. 1 ): Figure 1: Screening procedure for selection of polymers that support hESC culture. ( a ) Outline of the screening procedure used to select polymers that support hESC culture and passaging by thermodetachment. Cell attachment (nuclear count following DAPI stain), Oct3/4 and Nanog expression levels (immunocytochemistry) and thermodetachment ability (30 min at 15 °C) were assessed after culture of cells on polymer arrays. Successful polymers were selected for longer-term culture studies. ( b ) Cell detachment following lowering ambient temperature to 15 °C of hESC cultured on the top three polymers or Matrigel as control. Mean±s.d., n =3. ( c ) Chemical structure of polymers HG19, 20 and 21 with 1:3, 1:1 and 3:1 ratios of AEtMA-Cl/DEAEA, respectively. ( d ) Following thermodetachment of RH1 hESC from HG21 the majority of the remaining cells, visualized by DAPI-stained nuclei (blue) and phase-contrast light microscopy, are negative for Oct3/4 (green) and Nanog (red) (immunocytochemistry). Scale bar, 100 μm. ( e ) Cell growth curves of RH1 hESC cultured on HG21 or MG, plotted as mean fold increase (±s.e.m., n =3 biological replicates) relative to when cells were plated (day 0). *** P <0.001, **** P <0.0001 compared to D1. Full size image First, we selected the top 120 candidates, from two independent polymer screens, which supported cell attachment after 24 h, as determined by 4′,6-diamidino-2-phenylindole (DAPI)-positive nuclear staining ( Supplementary Fig. S2 ). This screen was followed by re-screening of top candidates selected from phase 1 for support of short-term culture of pluripotency-associated transcription factor marker positive hESC for 2, 4 and 7 days (growth data in Supplementary Figs S3 and S4 , and expression of Oct3/4 and Nanog in Supplementary Fig. S4 ). Last, the best 25 polymers were scaled up and tested as coatings on glass coverslips to evaluate their support of hESC attachment, viability and morphology over 7 days of culture, followed by assessment of the efficiency of thermal release by lowering the temperature to 15 °C for 30 min, gentle pipetting and subsequent cell replating ( Fig. 1b and Supplementary Fig. S5 ). The cumulative outcome of this effort was the identification of three polymers, henceforth called hydrogels (HG), HG19, HG20 and HG21 that were similar to or better than Matrigel for support of short-term attachment and growth of undifferentiated hESC as colonies over 7 days, and from which the majority of undifferentiated hESC colonies, but not spontaneously differentiating cells outside of colonies, could be released by thermomodulation ( Fig. 1d ). These three HGs formed part of a family that contained the monomers 2-(acryloyloxyethyl) trimethylammonium chloride (AEtMA-Cl) and 2-(diethylamino)ethyl acrylate (DEAEA) in varying ratios. HG21, consisting of AEtMA-Cl and DEAEA in a ratio of 3:1 ( Fig. 1c ) and providing as much as >90% reagent-free thermal release of cells at passaging ( Fig. 1b and Supplementary Movies 1 and 2 ) was selected based on performance, to assess competence to support long-term maintenance of hESC. HG21 supports hESC maintenance To characterize the ability of HG21 to support hESC maintenance, the RH1 hESC line was cultured continuously for more than 20 passages in mTeSR1 on HG21-coated glass coverslips. Undifferentiated hESC colonies were passaged by reducing the temperature to 15 °C for 30 min, followed by gentle pipetting without using any cell dissociation reagents to dislodge cell colonies from the HG substrate ( Supplementary Movie 1 ). Detachment of colonies yielded aggregates similar to those achieved with collagenase-mediated dissociation, which could be fully dissociated to single cells for further culture or analysis by brief (5 min) treatment with trypsin/EDTA at 37 °C if required. Real-time monitoring of shear force applied using a rheometer established that the force required for colony detachment ranged between 75 and 125 Pa, and was dependent on colony size, with larger colonies requiring more force ( Table 1 and Supplementary Movie 2 ). Table 1 Shear stress required for hESC detachment after temperature drop. Full size table Cells cultured on Matrigel could not be dislodged even when the shear force was increased to up to 154 Pa. The extent to which HG21-cultured cells remained attached to their matrix upon routine cell passaging also depended on the applied force. Typically, slow gentle pipetting (10–20 times) following thermomodulation resulted in detachment of the population to the extent that the remaining cells did not cover more than 5% of the total surface area ( Fig. 1b and data not shown). In situ immunocytochemistry (ICC) revealed that, with the exception of cells in small residual colonies, cells which remained attached were predominantly negative for Nanog and Oct3/4 and thus likely to be differentiating derivatives ( Fig. 1d ). In practice, RH1 hESC growth on HG21 appeared slower than observed on Matrigel. HG21 cultures routinely took 8–10 days to reach 80% confluence as opposed to 4–5 days for Matrigel, despite being plated at a higher pre-to-post plating ratio of 1:1.5 versus 1:2 wells, respectively. This was confirmed by measurement of cell growth over each of 5 days, which revealed a slower rate of expansion on HG21, and lower total expansion over 5 days from a mean (±s.e.m.) of 17.40-fold (±0.47) to 7.68-fold (±0.04) for Matrigel and HG21, respectively ( Fig. 1e ; P <0.0001). This equates to 4.2 versus 2.8 population doublings over this interval, and population doubling times of ~29 versus 43 h, respectively. There was no apparent increase in non-adherent cells in the medium of HG21-cultured cells compared with Matrigel. Interaction of HG21 with cell culture medium To assess whether HG21 could capture or release proteins in mTeSR1 medium, coated coverslips were cultured at 37 °C, followed by washing to remove unbound protein at 37 and 15 °C, and assessment of HG21 incorporated proteins by one-dimensional polyacrylamide gel electrophoresis and mass spectrometry ( Supplementary Methods ). HG21-captured proteins presented as seven discrete bands, the intensity of which for most (2–7) was significantly reduced after temperature reduction to 15 °C ( Fig. 2a ). Mass spectrometry analyses revealed that all bands represented fragments of bovine serum albumin (BSA; data not shown), a known component of mTeSR1 (ref. 2 ). 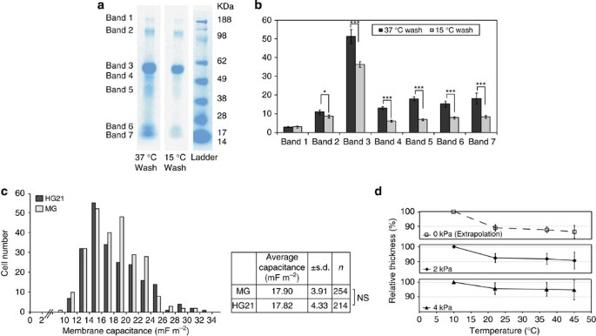Figure 2: Membrane capacitance of HG21-cultured hESC and physical properties of HG21. (a) Gelcode blue staining of 1-D polyacrylamide gel electrophoresis of proteins incorporated and retained in HG21 after incubation with mTeSR1 at 37 °C, followed by washing with PBS at 37 and 15 °C. Seven bands, ranging in size from ~17–188 kDa, were apparent under both conditions but less abundant in the latter. (b) Quantification of mean stained protein band intensity (±s.d;n=4) normalized to background confirmed significant reduction in the retention of most bands (2–7) in HG21 upon temperature reduction (Student’st-test, ***P<0.001; **P<0.01). (c) Long-term culture on HG21 does not significantly alter cell membrane biophysical properties from those observed for cells cultured on Matrigel (MG). Distribution and average cell membrane capacitance values for RH1 populations on HG21 and MG, as measured by dielectrophoresis. No significant difference was observed between cells grown on MG versus HG21 after 20 passages (two-tailedt-test, null hypothesis;P=0.8338). (d) Change in relative thickness of HG21 as a function of temperature in response to actual (2 and 4 kPa) and extrapolated (0 kPa) compressive forces, confirming swelling of HG21 at lower temperatures. NS, not significant. Figure 2: Membrane capacitance of HG21-cultured hESC and physical properties of HG21. ( a ) Gelcode blue staining of 1-D polyacrylamide gel electrophoresis of proteins incorporated and retained in HG21 after incubation with mTeSR1 at 37 °C, followed by washing with PBS at 37 and 15 °C. Seven bands, ranging in size from ~17–188 kDa, were apparent under both conditions but less abundant in the latter. ( b ) Quantification of mean stained protein band intensity (±s.d; n =4) normalized to background confirmed significant reduction in the retention of most bands (2–7) in HG21 upon temperature reduction (Student’s t -test, *** P <0.001; ** P <0.01). ( c ) Long-term culture on HG21 does not significantly alter cell membrane biophysical properties from those observed for cells cultured on Matrigel (MG). Distribution and average cell membrane capacitance values for RH1 populations on HG21 and MG, as measured by dielectrophoresis. No significant difference was observed between cells grown on MG versus HG21 after 20 passages (two-tailed t -test, null hypothesis; P =0.8338). ( d ) Change in relative thickness of HG21 as a function of temperature in response to actual (2 and 4 kPa) and extrapolated (0 kPa) compressive forces, confirming swelling of HG21 at lower temperatures. NS, not significant. Full size image Biophysical properties of hESC cultured on HG21 Next, dielectrophoresis (DEP) was performed to investigate whether culture on HG21 altered the biophysical properties of hESC and their membranes ( Supplementary Methods ). DEP can identify cellular states associated with cell activation, apoptosis and necrosis [27] . It discriminates distinct cellular identities in heterogeneous populations on the basis of single-cell polarity and membrane capacitance in an electrical field gradient. No difference in the distribution range or average membrane capacitance (two-tailed t -test, null hypothesis; P =0.8338) was observed between RH1 cells grown on Matrigel or HG21 (passage 20; Fig. 2c ). Characterization of physical properties of HG21 To determine how bound hESC were thermally detached, mechanical analyses of HG21 were performed ( Supplementary Methods ). The temperature-dependent alteration of the physical structure of HG21 was examined by rheology in phosphate-buffered saline (PBS) between 10 and 45 °C under constant compressive forces (2 or 4 kPa). Extrapolation to zero compressive force (the situation analogous to cell culture) showed that HG21 increased in relative thickness, when the temperature was reduced from 37 to 15 °C ( Fig. 2d ). Thus, at 37 °C HG21 allows the attachment and growth of hESC. After 30 min incubation at 15 °C HG21 becomes more hydrated, resulting in the detachment of cell colonies. Similar data were obtained for the two HGs, HG19 and HG20, that are composed of the same monomers as HG21 (but in different ratios), which affects HG thickness following a reduction in temperature ( Supplementary Fig. S6 ). Further analyses of HG21 to assess the expected properties of this HG showed that its storage modulus ( G ′) was much greater than the loss modulus ( G ″) in the measurement range of strain, a typical property of a HG network ( Supplementary Fig. S7 ) [28] , and X-ray photoelectron spectroscopy analysis confirmed the concordance between the actual and theoretical molecular composition of HG21 ( Table 2 ). Table 2 Theoretical and experimentally determined composition of HG21. Full size table Characteristics of hESC cultured on HG21 Similarly to culture on Matrigel, RH1 hESC on HG21 grew as colonies ( Fig. 3a ), which were positive for the pluripotency-associated transcription factors Nanog and Oct3/4 ( Fig. 3b ). Quantitative reverse transcription-PCR (qPCR) confirmed that RNA levels of these transcription factors, in addition to another pluripotent cell transcription factor, Sox2, were similar to respective Matrigel controls ( Fig. 3c ). Fluorescence activated cell sorting (FACS) of HG21-cultured RH1 cells for pluripotent cell-associated surface markers also confirmed high expression of SSEA-4 and TRA-1-60R, and low expression of SSEA-1 ( Fig. 3d ). Functional pluripotency to form tissues representative of all three germinal lineages was confirmed by both embryoid body (EB)-mediated differentiation in vitro ( Fig. 3e ) and teratoma formation in vivo following injection under the kidney capsule of immunodeficient mice ( Fig. 3f ). Comparative genome hybridization (CGH) analysis using a Nimblegen 135 k probe whole genome tiling array, with a median probe spacing of 12,524 base pairs ( Supplementary Methods ), did not reveal any copy number variations in HG21-cultured cells, which were not also apparent following growth on Matrigel. However, microdeletions and duplications ranging from 0.5 to 1.5 Mb were apparent under both culture conditions on chromosomes 8, 9, 13 and 20 ( [29] , [30] , [31] Fig. 3g , Supplementary Table S1 ). 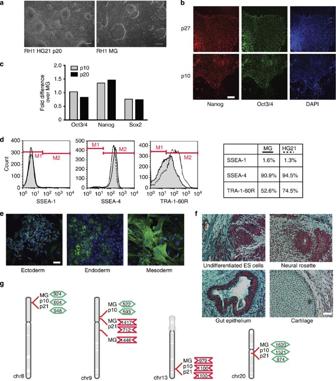Figure 3: Characterization of RH1 hESC cultured on thermomodulatable HG21. (a) Representative micrographs of hESC colonies cultured on HG21 (left) and Matrigel (MG, right). Scale bar, 100 μm. (b) Immunocytochemistry (ICC) for Nanog (red) and Oct3/4 (green) expression in RH1 hESC cultured on HG21 for 10 and 27 passages. Scale bar, 100 μm. (c) qPCR analysis of RNA expression of the pluripotency markers Oct3/4, Nanog and Sox2 for RH1 hESC cultured on HG21 for 10 and 20 passages. Expression levels were normalized to glyceraldehyde 3-phosphate dehydrogenase, and data represented as fold-change compared with expression in MG-cultured RH1 hESC. Data are representative examples of minimally two independent qPCR experiments per gene. (d) SSEA-1, SSEA-4 and TRA-1-60R cell surface markers are expressed at similar levels on RH1 hESC cultured on HG21 (dashed line) and MG (solid line, grey area), as determined by flow cytometry. M1 and M2 gates discriminate background to signal fluorescence thresholds. Apposing table depicts cell percentages with fluorescence signal intensity above background. (e) After 20 passages on HG21, RH1 hESC can differentiate to all three germ layers, as shown by ICC for β-tubulin III (ectoderm; green), α-fetoprotein (endoderm; green) and α-smooth muscle actin (mesoderm; green). Nuclei were stained with DAPI (blue). Scale bar, 20 μm. (f) Kidney capsule teratomas, induced by injection of RH1 hESC cultured for 20 passages on HG21 into NOD/SCID mice, contain tissue derived from all three primary germ layers. Clockwise: islands of undifferentiated EC/ES cells, neural rosettes (ectoderm), gut epithelium (endoderm) and cartilage (mesoderm). (Masson’s trichrome stain). Scale bar, 100 μm. (g) Schematic summary of gene variations detected by CGH analysis of RH1 hESC using a NimblegenTM 135 K probe array following culture on HG21 for 10 and 21 passages (p10, p21) and age-matched MG (MG) (21 passages). Depicted are microdeletions and insertions (>no.<,<no.>, respectively, and their size in kilobase pairs) in relation to their location on chromosomes per genomic DNA sample. No gross chromosomal aneuploidies were detected between HG21 and MG-grown cells. Copy number variations occurring in the former also occurred in the latter on chromosomes 8, 9, 13 and 20. Figure 3: Characterization of RH1 hESC cultured on thermomodulatable HG21. ( a ) Representative micrographs of hESC colonies cultured on HG21 (left) and Matrigel (MG, right). Scale bar, 100 μm. ( b ) Immunocytochemistry (ICC) for Nanog (red) and Oct3/4 (green) expression in RH1 hESC cultured on HG21 for 10 and 27 passages. Scale bar, 100 μm. ( c ) qPCR analysis of RNA expression of the pluripotency markers Oct3/4, Nanog and Sox2 for RH1 hESC cultured on HG21 for 10 and 20 passages. Expression levels were normalized to glyceraldehyde 3-phosphate dehydrogenase, and data represented as fold-change compared with expression in MG-cultured RH1 hESC. Data are representative examples of minimally two independent qPCR experiments per gene. ( d ) SSEA-1, SSEA-4 and TRA-1-60R cell surface markers are expressed at similar levels on RH1 hESC cultured on HG21 (dashed line) and MG (solid line, grey area), as determined by flow cytometry. M1 and M2 gates discriminate background to signal fluorescence thresholds. Apposing table depicts cell percentages with fluorescence signal intensity above background. ( e ) After 20 passages on HG21, RH1 hESC can differentiate to all three germ layers, as shown by ICC for β-tubulin III (ectoderm; green), α-fetoprotein (endoderm; green) and α-smooth muscle actin (mesoderm; green). Nuclei were stained with DAPI (blue). Scale bar, 20 μm. ( f ) Kidney capsule teratomas, induced by injection of RH1 hESC cultured for 20 passages on HG21 into NOD/SCID mice, contain tissue derived from all three primary germ layers. Clockwise: islands of undifferentiated EC/ES cells, neural rosettes (ectoderm), gut epithelium (endoderm) and cartilage (mesoderm). (Masson’s trichrome stain). Scale bar, 100 μm. ( g ) Schematic summary of gene variations detected by CGH analysis of RH1 hESC using a NimblegenTM 135 K probe array following culture on HG21 for 10 and 21 passages (p10, p21) and age-matched MG (MG) (21 passages). Depicted are microdeletions and insertions (>no.<,<no.>, respectively, and their size in kilobase pairs) in relation to their location on chromosomes per genomic DNA sample. No gross chromosomal aneuploidies were detected between HG21 and MG-grown cells. Copy number variations occurring in the former also occurred in the latter on chromosomes 8, 9, 13 and 20. Full size image HG21 supports multiple hESC lines To confirm the ability of HG21 to support the continuous culture of other hESC lines, HG21 was evaluated for the support of H9 hESC over 5–10 passages. In practice, cultivation of H9 cells on HG21 was as for RH1, taking longer to achieve confluence than H9 on Matrigel despite seeding at a higher pre-to–post plating ratio (1:1.5 versus 1:2). Assessment of H9 hESC after six passages confirmed comparable expression of pluripotency-associated markers by immunocytochemistry (ICC; Oct3/4 and Nanog) and qPCR (Oct3/4, Nanog, Sox2) ( Supplementary Fig. S8 ). After nine passages injection into immunodeficient mice yielded teratomas with tissues representative of three germinal lineages, supporting preservation of pluripotency ( Supplementary Fig. S8 ). CGH analysis of H9 cells grown on HG21 and Matrigel at this time also revealed no major chromosome aneuploidy. H9 grown on either substrate possessed a micro-duplication of 0.5 Mb on chromosome 20 in common with RH1, and different micro-duplications and deletions on chromosomes 14 and 16 associated with one or the other culture conditions, not observed in RH1 ( Supplementary Table S1 ). Characterization of hESC attachment to HG21 To understand the basis of hESC attachment to HG21, we evaluated the expression profiles of cell surface proteins known to mediate cell–matrix interactions, for both RH1 and H9 hESC lines on HG 21 and Matrigel by flow cytometry and/or ICC. This included analysis of E-cadherin, epithelial cell adhesion molecule (EpCAM), α-integrins 1–6 and v, β-integrin 1 and 2, and three α/β integrin heterodimers (α5β1, αvβ3 and αvB3). Antibody probes which provided conclusive results for flow cytometry (α1–6, β1, E-cadherin, EpCAM) and ICC (all but α1, E-cadherin and EpCAM) revealed comparable expression of cell adhesion molecules for both cell lines on both matrices, with integrin α4 being the least prevalent of those that were detected by flow cytometry ( Fig. 4 , Supplementary Figs S9 and S10 ). To confirm the role for integrins in cell attachment to HG21, RH1 and H9 hESC were incubated with known integrin heterodimer-blocking antibodies (α5β1 or αvβ3) or, as a positive control, a cocktail of all integrin antibodies used for characterization, while in suspension before plating and after plating ( Supplementary Methods ). Following culture for 4–18 h neither of the two integrin heterodimer-blocking antibodies affected attachment to either HG21 or Matrigel ( Supplementary Fig. S11 ). In contrast, the pan-integrin antibody cocktail interfered with adherence of hESC colonies to both HG21 and Matrigel, resulting in cells in suspension singly and as clusters of loosely and densely packed cells, the latter resembling EB-like structures. (Shown for H9, Supplementary Fig. S11 ). Treatment with the divalent cation chelating agent EDTA (2.5 mM in mTeSR1) also blocked cell attachment to both substrates (Shown for H9, Supplementary Fig. S11 ). 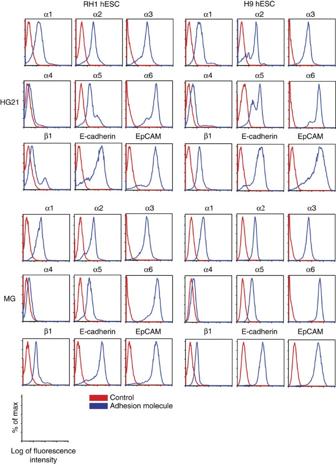Figure 4: Analyses of hESC adhesion molecule expression. RH1 (left panel sets) and H9 (right panel set) hESC cultured on HG21 (top panel sets) and Matrigel (MG, bottom panel sets) possess similar expression profiles for integrins α1–6, β1, EpCAM and E-cadherin, as assessed by flow cytometry. Vertical axis, percentage of maximum cell counts on a linear scale. Horizontal axis, fluorescence intensity on a log scale for control background (red) and adhesion molecule specific (blue) signal. Figure 4: Analyses of hESC adhesion molecule expression. RH1 (left panel sets) and H9 (right panel set) hESC cultured on HG21 (top panel sets) and Matrigel (MG, bottom panel sets) possess similar expression profiles for integrins α1–6, β1, EpCAM and E-cadherin, as assessed by flow cytometry. Vertical axis, percentage of maximum cell counts on a linear scale. Horizontal axis, fluorescence intensity on a log scale for control background (red) and adhesion molecule specific (blue) signal. Full size image A number of synthetic substrates supportive of human pluripotent stem cell growth and pluripotency in long-term culture have been reported [11] , [13] , [14] , [15] , [16] , [32] , most of which rely on mechanical dissection at passaging. Though this type of passaging is a favoured means to preserve cell–cell associations important for promoting self-renewal and genetic stability, it is not tractable in large-scale and robotic culture systems. Proteolytic enzymatic digestion using collagenase, and chemically mediated chelation of divalent cations using EDTA represent pragmatic alternatives to dissociate cells as aggregates [13] , [17] . These methods are more amenable to high-throughput cell culture but still constitute aggressive disruptions of cell–cell and cell–substrate interactions. In addition, they also rely on transient exposure of cells to media and buffers other than the ones in which they are cultured. The thermoresponsive HG (HG21) and related polymers we report here overcome these limitations by providing a gentle method of passaging human pluripotent stem cells. They also enables separation of undifferentiated cell colonies from differentiating cells that remain attached. Prolonged culture on and adaptation to the HG21 substrate did not detectably affect the character of the cell membrane or its interaction with the substrate, as assessed by dielectrophoretic analysis of membrane capacitance. Most importantly, pluripotency was preserved and the cells did not appear to have adapted by the accumulation of chromosomal aneuploidies. Growth on HG21 was slower than on Matrigel, which might be a reflection of the stimulatory effect of the extracellular matrix components in the latter, including residual growth factors [33] . The absence of these factors in our HGs suggests that either the topography or reactive groups they provide for cell attachment provides sufficient mimicry of a biological substrate to support renewal, at least under the conditions of our study. To our knowledge there is no evidence that slower growth is detrimental to human pluripotent stem properties. In fact, typically it is accelerated growth that is associated with genetic mutation presumed to confer a growth advantage to subpopulations of cells that then come to dominate the culture [34] , [35] . We and others have reported the suitability of thermoresponsive polymers for mouse embryonic stem cell culture [25] , [36] . Loh et al . [36] observed reduced growth rates when culturing mouse embryonic stem cells on thermoresponsive co-polymers compared with gelatin controls. Although they demonstrated that these gelatin-containing polymers support mouse embryonic stem cell growth and cell release at very low temperature (4 °C), cell cultures lasted only 3–4 days, without cell passaging. To our knowledge, our study is the first to report long-term culture and gentle serial passaging of hESCs using a thermomodulatable synthetic polymer, verified with independent cell lines. Plasma treatment of plastic surfaces [37] followed by simple addition of the appropriate monomers permitted HG polymer coating of conventional plasticware. This surface substrate should therefore be readily applicable in the future to scaled production of hESC in automated systems for industrial and clinical purposes. It is now accepted that like any other cell in culture, hESC acquire non-random chromosomal aberrations during the course of culture adaptation. In hESC these particularly affect chromosomes 12, 17 and X, similar to aneuploidies observed in germ cell tumours [34] , [35] , [38] . These were not observed in our hESC cultured on Matrigel or HGs. Using CGH we did observe deletions and duplications as expected [34] , [35] ranging in size from 0.5 to 1.5 Mb on chromosomes 8, 9, 13 and 20 in cells cultured on both HG21 and those grown in control conditions. The appearance of the same small changes in both conditions strongly suggests that they were a feature of the cell lines themselves and not a culture adaptation specifically prompted by growth on a thermoresponsive substrate. One of the affected regions was an amplicon on chromosome 20q11.21, which has been associated with adaptation to culture conferring a growth advantage [31] . However, to date there are no reports that such an adaptation would undermine the differentiation potential of cells, and our data presented here confirm that the cells retain their undifferentiated state and pluripotency. Investigation of the mechanism of hESC attachment to HG21 confirmed similarities in cell adhesion molecule expression to cells grown on Matrigel, and conservation across two independent cell lines. Consistent with previous studies [13] , [14] , [15] , [17] , cell adhesion to both substrates was divalent cation and multi-integrin dependent. We observed that BSA and fragments in mTeSR1 incorporate into HG21 at 37 °C and are released at 15 °C. Serum- and serum protein-dependent hESC adhesion to substrates has been previously reported [9] , [10] , [11] and dependence of HG21 on serum albumin and other proteins is a subject of ongoing investigation. In this study, attempts to interfere with cell adhesion by exposure to known blocking antibodies to single integrin heterodimers (α5β1 or αvβ3) were not successful on either substrate, whereas exposure to a complex cocktail of cell adhesion molecule antibodies was. This is in line with findings by Mei et al . [13] who showed that simultaneous blocking of a selection of integrins had a more pronounced effect on abrogating adhesion of hESC to a matrix than the blocking of single integrins, thereby highlighting the redundancy for integrins in mediating adhesion of hESC to substrates. HG swelling induced by thermoreduction was in itself not sufficient to release undifferentiated hESC colonies, which still required gentle shearing forces provided through slow pipetting. Our interpretation therefore is that gel hydration only serves to destabilize interactions between cell adhesion molecules and polymer reactive groups. In conclusion, our study identifies and validates the utility of a chemically defined and thermomodulatable xeno-free substrate for the support of pluripotent hESC growth in long-term culture. The thermoresponsiveness of this substrate obviates alternative methods for cell passaging that can be damaging to cells and difficult to implement in scaled up and/or automated production. Collectively, these features substantiate the prospective merit of this substrate for pluripotent stem cell manufacture for banking, screening and therapeutic purposes. Materials Unless otherwise stated, cell culture reagents were sourced from Invitrogen. HG microarray fabrication chemicals were purchased from Sigma-Aldrich or ABCR GmbH Co.KG (tridecafluoro-1,1,2,2-tetrahydrooctyl-dimethylchlorosilane). N -acryloyl- N′ -propylpiperazine and 2,2′-(ethylenedioxy)bis(ethylamine) mono-acylamide were synthesized in-house, whereas N -isopropylacrylamide was purified by recrystallization as described previously [24] , [25] . Monomers are listed in Supplementary Table S1 . HG-coated coverslips for upscaling HG-coated coverslips and slides were prepared as follows: solutions of the monomers, crosslinker and photoinitiator in N -methyl-2-pyrrolidone were coated on 3-(trimethoxysilyl)propyl methacrylate-treated coverslips ( φ 13 mm, φ 19 mm and φ 32 mm), exposed to 365-nm UV light for 30 min to initiate polymerization, placed overnight in a 50 °C oven, washed with ethanol and acetone, and air dried. [25] hESC culture The use of hESC lines in this project was approved by the MRC steering committee overseeing the UK Stem Cell Bank. RCM1 (ref. 39 ) hESC and RH1 (ref. 40 ) hESC were derived at the Roslin Institute under a licence from the Human Fertilisation and Embryology Authority to P.A. de Sousa and licenced from Roslin Cells and Geron, respectively. Both lines have been deposited in the UKSCB ( www.ukstemcellbank.org.uk ). H9 hESC was licensed from WiCell (available from the Wisconsin International Stem Cell Bank ( www.wicell.org )) [41] . Starting cell populations for all three lines used here were at passage 60–70. All feeder-independent cultures were grown in mTeSR1 medium (STEMCELL Technologies) containing 50 U ml −1 penicillin, 50 μg ml −1 streptomycin and 2.5 μg ml −1 Fungizone (hereafter referred to as mTeSR1+P/S/Fgz) at 37 °C, 5% CO 2 , as reported previously [2] . hESC control cultures were grown on Matrigel (Becton Dickinson) and routinely passaged by mechanical scraping following treatment with collagenase IV (200 digestive units per ml in knockout DMEM). Cells were seeded at a density of ~100,000 cells cm −2 and split at a pre-to-post plating ratio of 1:2 wells. Cultures were passaged at 80% confluence every 4–5 days. hESC culture on polymer arrays Polymer arrays were screened using RCM1 hESC. Cells were dissociated with trypsin (0.25 g l −1 )/5 mM EDTA (T/E) at 37 °C to obtain single cells, which were plated (60,000 cells cm −2 ) on microarray slides in mTeSR1+P/S/Fgz containing 10 μM ROCK inhibitor (Calbiochem). Cells were incubated for 2, 4 or 7 days in mTeSR1+P/S/Fgz before fixation in 4% paraformaldehyde in PBS for cell staining. hESC culture on polymer-coated glass surfaces Polymer-coated coverslips were placed in tissue culture plate wells. After sterilizing, plates (20 min under UV light) wells were washed with PBS and cells seeded (90,000 cells cm −2 ). Cells were split at a pre-to-post plating ratio of 1:1.5 wells. Cultures were passaged at 80% confluence every 8–10 days. Thermodetachment was achieved by incubation at 15±3 °C for 30 min. Cell aggregates originating from thermodetached colonies were resuspended in fresh mTeSR1+P/S/Fgz and replated. Cells were maintained by daily replacement of the medium with fresh mTeSR1+P/S/Fgz equilibrated to 37 °C. Assessment of temperature-mediated cell detachment To quantify temperature-mediated detachment of cells grown on HG21 versus Matrigel, the percentage of cells that detached following temperature reduction was calculated as follows: after placing the culture plates at 15 °C for 30 min, detached cells were harvested, treated with T/E to obtain a single-cell suspension, and counted after Trypan blue staining using a haemocytometer (=Fraction A). The remaining cells were dissociated from the wells by trypsinization and counted (=Fraction B). The percentage of thermodetached cells were calculated as follows: Fraction A/(Fraction A+B) × 100% ( n =3). To measure the (minimal) shear stress required to detach cells from HG21, hESC were cultured for 4 days in Φ35 Petri dishes that were either directly coated with Matrigel or contained an HG21-coated coverslip (glued to the bottom). At day 4, Petri dishes were incubated for 30 min at 15°C before shear stress analysis, which was performed using a TA AR2000 rheometer with a spinning cone (Φ20 mm, 4°, a truncation gap of 92 mm between cone and the Petri dish surface) to generate a controlled culture medium flow to detach adherent cells. Movies of this detachment were recorded with a homemade imaging module with an × 10 objective in reverse mode, a light-emitting diode light source, and a charge-coupled device camera (0.16 × 0.16 micrometre pixel) ( Supplementary Movie 2 ). Visualization of hESC thermodetachment from HG21 without shear force analysis was performed using a Debut Video Capture system attached to an Infinity 2 Meiji TC 5600 microscope ( Supplementary Movie 1 ). Immunostaining Cells on glass coverslips coated with either HG21 or Matrigel were stained using standard immunocytochemistry protocols. hESC were fixed with 4% PFA, incubated overnight with primary antibodies against stem markers (Oct3/4 (Santa Cruz Biotechnology), Nanog (R&D systems), β3-tubulin (Sigma), AFP (Sigma) and α-smooth muscle actin (DAKO)) or against a selection of integrins (Chemicon kit ECM435 and Millipore kit ECM430; all antibodies used at 1/500), and incubated with appropriate Alexafluor-conjugated secondary antibodies (Invitrogen). Nuclei were labelled using DAPI. Imaging was performed with a Leica SPE or Zeiss Observer microscope. Flow cytometric analysis of population size To obtain population growth curves, cells grown for 1−5 days on HG21-coated coverslips or on Matrigel in 12-well tissue culture plates (in triplicate) were harvested on consecutive days using T/E (5 min at 37 °C). Following quenching (PBS/10% FCS) cells were washed, incubated with 60,000 fluorspheres (Flow-check Fluorspheres, Beckman Coulter) per sample in ice-cold PBS/0.1% BSA and immediately acquired with a FACSCalibur flow cytometer counting 5,000 fluorspheres per sample. Data were analysed and plotted as fold increase over the cell number at the day of plating (D0), using GraphPad Prism software. Quantitative reverse transcription-PCR hESC RNA was prepared from snap-frozen cell pellets using TRIzol Reagent (Invitrogen) according to manufacturer’s instructions. cDNA was prepared using a SuperScript 3 reverse transcription kit with oligo-dT as primers. After confirmation of negligible genomic DNA contamination (PCR amplification of human glyceraldehyde 3-phosphate dehydrogenase from cDNA generated in reverse transcription reaction containing no reverse transcriptase) qPCR was performed using SYBR green on a BioRad CFX96 C1000 thermo-cycler. Primer sequences and annealing temperatures are listed in Supplementary Table S2 . Three technical replicates were amplified for each sample, with minimally two independent qPCR experiments per gene. Replicates where CT values deviated from others by more than 0.5 were excluded from analysis and experiments repeated in their entirety if two CT values for a sample had to be discarded by this criterion. Results were normalized relative to housekeeping gene glyceraldehyde 3-phosphate dehydrogenase by the ΔΔCT relative method [42] . Flow cytometric analysis of cell surface markers Following matrix-appropriate cell detachment (thermodetachment for HG21, and collagenase IV treatment followed by mechanical scraping for Matrigel) cells were washed, dissociated by incubation with T/E (5 min at 37 °C), washed (PBS/5% FCS) and resuspended in PBS/0.1% BSA. To assess stemness, cells were incubated with FITC-labelled anti-SSEA-4, phycoerythrin-labelled anti-SSEA-1, and biotinylated anti-TRA-1-60R (all Biolegend) in PBS/0.1% BSA for 30 min on ice. Tra1-60R biotin was detected with streptavidin-conjugated Allophycocyanine (Biolegend). To assess integrin expression, cells were incubated with a panel of fluorescently labelled anti-integrin antibodies (α1–6, β1 and EpCAM; all BD) (singly stained; 1/50 in PBS/0.1% BSA) for 30 min on ice. Data were acquired with a FACSCalibur flow cytometer (Becton Dickinson) and analysed using FlowJo software. Per condition data for at least 30,000 live cells were collected. Gating was set relative to unstained controls from the same cell population. EB-mediated differentiation EB-mediated differentiation was achieved as previously described [39] , [43] . In short, cells were grown in suspension for 7 days at 37 °C, 5% CO 2 in EB medium (DMEM, 20% fetal calf serum (Sigma), 2 mM L -Glutamine, 100 nM NEAA, 0.1 mM 2-mercaptoethanol (Sigma)), after which EBs were dissociated in PBS-based enzyme-free cell dissociation solution (Sigma) for 10 min at 37 °C and plated on Matrigel in EB medium plus 10 μM ROCK inhibitor (Calbiochem) overnight. To steer cells towards endoderm, ectoderm and mesoderm, cells were subsequently incubated for 6 days at 37 °C, 5% CO 2 in EB differentiation medium (advanced RPMI-1640, B27 supplement, 50 U ml −1 penicillin, 50 μg ml −1 streptomycin and 2.5 μg ml −1 Fungizone) in the presence of differentiation factors, as described [43] , with the exception that ectoderm was obtained by incubating the cells in the presence of 1 μM retinoic acid instead of Noggin. Teratoma induction RH1 hESC grown on HG21 were resuspended at 5 × 10 7 cells ml −1 in HEPES-buffered DMEM medium. Twenty microlitres of this cell preparation was placed under kidney capsules of anesthetized NOD/SCID mice (NOD.CB17-Prkdc-scid/J, Jackson Laboratories) ( n =6) using a fine glass capillary. Upon detection of teratomas, at least 4 weeks post injection, mice were culled and teratomas dissected, fixed overnight (10% phosphate-buffered formalin) and embedded in paraffin. Sections were stained with Masson’s Tricolour stain. Mice were housed in specific pathogen-free conditions and procedures were in accordance with UK home office regulations. For HG21-grown H9 hESC, teratomas were generated by the injection of cells into testes of narcotized fox chase SCID beige mice (1.2 × 10 6 cells per animal). After 5 weeks, mice were euthanized, and teratomas dissected, fixed overnight (4% PFA), and prepared for haematoxylin and eosin staining. How to cite this article: Zhang, R. et al . A thermoresponsive and chemically defined hydrogel for long-term culture of human embryonic stem cells. Nat. Commun. 4:1335 doi: 10.1038/ncomms2341 (2013).